Arrays of giant octagonal and square cylinders by liquid crystalline self-assembly of X-shaped polyphilic molecules Nanopatterning by molecular self-assembly has been a topic of intense research in pursuit of 'bottom-up' methods of generating structures for use in nanotechnology. The systems most widely studied have been two- and three-dimensional morphologies of block copolymers. However, T- and X-shaped polyphilic liquid crystals have recently been shown to have great potential for generating soft honeycomb-like structures, surpassing those of polymers in both complexity and degree of order. The cell cross-section of the liquid crystals honeycombs has so far been limited by small molecular size. Here we overcome this limitation by exploiting the inability of the polyphiles to simultaneously achieve optimal packing and complete nanophase separation. This frustration results in a two-dimensional periodic honeycomb consisting of giant octagonal and square cylinders with circumferences of 12 and 8 molecules, respectively. In addition to forming large cells, the two-molecule-long bendy walls give this structure extra versatility and stability. Creation of complexity in self-organized chemical systems is of acute interest for structuring surfaces [1] , [2] , [3] , [4] , [5] , templating solid-state structures and obtaining soft materials with new functionalities [6] , [7] , [8] , [9] . In the field of soft matter engineering, block copolymers have provided a variety of complex and hierarchically organized morphologies [10] , [11] , [12] , [13] . However, in recent years there has also been significant progress in increasing the complexity of self-assembly in low-molecular-weight supramolecular systems [14] , [15] , [16] , [17] and in liquid crystalline (LC) materials [18] , [19] , [20] , [21] . T-shaped [22] , [23] and X-shaped [24] block molecules ( Fig. 1a ) bearing up to four types of mutually incompatible groups A–D (tetraphilic) were found to form many new types of fluid self-assembled structures, among them a series of polygonal honeycombs [21] , [25] , [26] . In these honeycombs, the π-conjugated rod-like cores (B) form cell walls connected at the 'seams' by terminal hydrogen-bonding groups (A). The honeycomb cells of polygonal cross-section and infinite length are filled with the fluid lateral chains C for T-shaped molecules, or C+D for X-shaped molecules. Depending on the ratio of the volume of C+D to the length of the rod (2A+B), cells ranging from triangular to hexagonal were obtained [21] , [25] , [26] . Projected on an Euclidian plane, these honeycombs can be described as periodic tiling patterns [21] , [23] . Where chains C and D are different and incompatible, honeycombs are formed with cells filled with different material (C or D). These honeycombs can be considered as two-colour tiling patterns [25] , [26] . Previously reported two-colour tilings with trigonal and hexagonal symmetry are shown in Fig. 1b–d [25] , [26] . 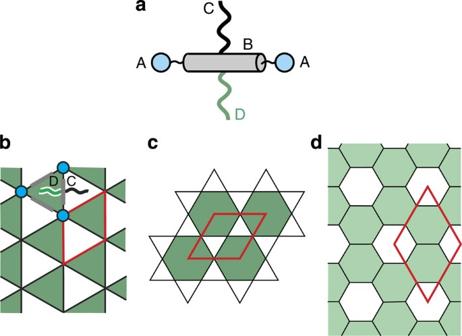Figure 1: Two-colour honeycombs in tetraphilic LC compounds. (a) Schematic molecular structure of an X-shaped polyphile. (b–d) Examples of two-colour honeycombs (cross-sections perpendicular to the columns)25,26. The light-green cells indcontain an approximately 3:1 mixture of D and C. Figure 1: Two-colour honeycombs in tetraphilic LC compounds. ( a ) Schematic molecular structure of an X-shaped polyphile. ( b–d ) Examples of two-colour honeycombs (cross-sections perpendicular to the columns) [25] , [26] . The light-green cells in d contain an approximately 3:1 mixture of D and C. Full size image In most cases, the length of the sides of the polygon (triangle, hexagon and so on) is one molecule, thus limiting the cylinder size. In the present work, we show how X-shaped molecules with two different side chains can form highly ordered honeycombs of giant square and octagonal cells, whose circumference contains not just 4 and 8, but 8 and 12 molecules, respectively, arising through the interplay between frustrations in both space-filling and microphase separation. The resulting large-cell honeycombs present a new level of complexity in self-assembled soft matter. The new phase in compounds 1 Herein, a new two-colour tiling pattern is reported, having the relatively rare square symmetry and combining two different types of cylinders. Compounds 1a – 1d (see Table 1 ) forming this new LC phase, were synthesized as described in the Methods and Supplementary Methods ( Fig. 5 ); the differential scanning calorimetry (DSC) traces are shown in Supplementary Figs S1–S4 . In these compounds, an aliphatic hydrocarbon chain ( C = R H ) and a semiperfluorinated chain, comprising a C 12 F 25 segment ( D = R F ), were attached laterally at opposite sides of a rod-like p -terphenyl core (B). To each of its ends, a glycerol groups (A) was attached, capable of forming a cooperative and dynamic hydrogen-bonding network. Hence, these compounds represent Janus -type [27] , [28] , [29] , [30] , [31] , [32] , [33] X-shaped quaternary amphiphiles. An equivalent series of compounds 2 was also synthesized, having a shorter C 10 F 21 segment instead of the C 12 F 25 segment. Only a representative example 2a ( Supplementary Fig. S5 ) is included in Table 1 for comparison with compounds 1 ; the complete 2 series will be described in detail elsewhere. Table 1 Transition temperatures, associated enthalpies* and lattice parameter of compounds 1a – 1d and 2a . Full size table Figure 5: Synthesis of compounds 1a – 1d and 2a . Reagents and conditions: ( i ) Br 2 , AcOH, 20 °C, 1 h; ( ii ) BnCl, K 2 CO 3 , MeOH, reflux, 30 min; ( iii ) C n H 2 n +1 Br, K 2 CO 3 , CH 3 CN, reflux, 6 h; ( iv ) Pd(PPh 3 ) 4 , NaHCO 3 , glyme, reflux, 10 h; ( v ) H 2 , Pd/C, EtOAc, 45 °C, 3.2 bar, 8 h; ( vi ) C m F 2 m +1 (CH 2 ) 6 Br ( m =10, 12), K 2 CO 3 , dimethylformamide, 80 °C, 6 h; and ( vii ) HCl, MeOH, reflux, 6 h. Full size image As shown in Table 1 , all compounds 1a – 1d form enantiotropic (thermodynamically stable) LC phases in a 21 to 38 K wide temperature range between the crystalline and the isotropic liquid states. Compounds 1c and 1d form only one LC phase (Col squ / p 4 gm) , whereas an additional, still unknown, mesophase (M) is found in compounds 1a and 1b in a very narrow range just below the isotropization temperature. 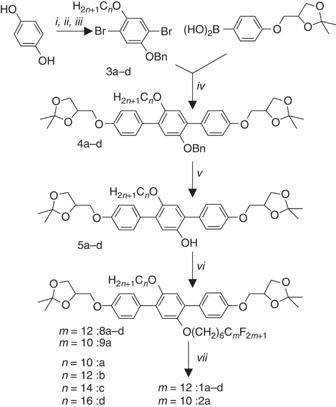Figure 5: Synthesis of compounds1a–1dand2a. Reagents and conditions: (i) Br2, AcOH, 20 °C, 1 h; (ii) BnCl, K2CO3, MeOH, reflux, 30 min; (iii) CnH2n+1Br, K2CO3, CH3CN, reflux, 6 h; (iv) Pd(PPh3)4, NaHCO3, glyme, reflux, 10 h; (v) H2, Pd/C, EtOAc, 45 °C, 3.2 bar, 8 h; (vi) CmF2m+1(CH2)6Br (m=10, 12), K2CO3, dimethylformamide, 80 °C, 6 h; and (vii) HCl, MeOH, reflux, 6 h. Here we focus on the major phase, denoted Col squ / p 4 gm . The optical texture, as observed between crossed polarizers, is characterized by 'spherulitic' domains combined with regions appearing completely dark, where the optic axis is normal to the LC film (homeotropic regions), see Fig. 2a . These textures indicate an optically uniaxial columnar LC phase. The samples are easily sheared; this destroys the homeotropic texture converting it to a nonspecific birefringent one, indicating the fluidity of the material. Lack of atomic-scale order is additionally confirmed by the diffuseness of the wide-angle X-ray scattering (see inset in Fig. 2c and Supplementary Fig. S6 ). Incidentally, the position of the diffuse maximum corresponds to a Bragg spacing of 0.54 and 0.53 nm for compounds 1a and 1b , respectively, as the proportion of the perfluorinated segment diminishes, dropping to 0.46 nm for related compounds with no fluorination [24] . The small-angle Bragg reflections ( Fig. 2c and Supplementary Fig. S7 ) of all four compounds can be indexed on a square lattice with p 4 gm plane group symmetry (Col squ / p 4 gm phase) and lattice parameters ranging between 9.37 and 9.83 nm, increasing with increasing alkyl chain length ( Table 1 and Supplementary Tables S1–S4 ). Indexing was facilitated by grazing-incidence small-angle X-ray scattering (GISAXS) on aligned thin films ( Fig. 2d ; Supplementary Fig. S8 ). The orientation of the π-conjugated aromatic cores is deduced from the colour of the fans in the micrograph taken with a λ-plate ( Fig. 2b ). The directions of yellow and blue fans with respect to the indicatrix of the retarder confirm the orientation of the high-index axis as radial to the fans. 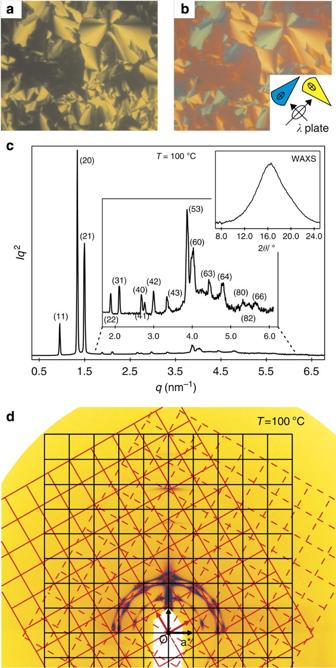As the columns are tangential and the high-index axis is parallel to the terphenyl long axis, it follows that the terphenyls are perpendicular to the column long axis, which is typical for polygonal honeycomb structures. Figure 2: Thep4gmphase of compounds 1. (a) Optical texture of compound1aatT=110 °C (crossed polarizers). (b) Same texture, but with λ-retarder plate (the indicatrix orientation in the compensator is shown on the right). (c) SAXS pattern of thep4gmphase of1aat 100 °C; the inset is theθ-scan of the diffraction pattern of1ain the wide-angle region, recorded with CuKαradiation. (d) GISAXS pattern of thep4gmphase of1bat 100 °C; superimposed are reciprocal lattices for two of the observed orientations, with (10) and (21) planes in contact with the substrate, respectively (([macr2]1) orientation with dashed lines); pattern showing (11) orientation is shown inSupplementary Fig. S8. Figure 2: The p 4 gm phase of compounds 1. ( a ) Optical texture of compound 1a at T =110 °C (crossed polarizers). ( b ) Same texture, but with λ-retarder plate (the indicatrix orientation in the compensator is shown on the right). ( c ) SAXS pattern of the p 4 gm phase of 1a at 100 °C; the inset is the θ -scan of the diffraction pattern of 1a in the wide-angle region, recorded with CuK α radiation. ( d ) GISAXS pattern of the p 4 gm phase of 1b at 100 °C; superimposed are reciprocal lattices for two of the observed orientations, with (10) and (21) planes in contact with the substrate, respectively (([macr2]1) orientation with dashed lines); pattern showing (11) orientation is shown in Supplementary Fig. S8 . Full size image Hexagonal honeycomb in compounds 2 To provide the context for the new phase, we present briefly the relevant results for compound 2 . The second reason for presenting selected data on compounds 2 is that, because of their simple but related structure, they provide information on molecular area that will be used below to verify the proposed new structure in compounds 1 . Compounds 2a – d ( n =10–16) differ from compounds 1 only in having 10 rather than 12 fluorinated-end carbons in the R F chain ( Table 1 , m =10). These compounds only form the simple hexagonal honeycomb phase, Col hex with p 6 mm symmetry—see evidence in Supplementary Fig. S9 for compound 2a . Based on X-ray diffraction data ( Supplementary Fig. S9a and Supplementary Table S5 ), the electron density (ED) map is reconstructed for this compound and shown in Fig. 3a . Schematic molecules are superimposed. The model is supported by the fact that the length of a wall (the side of the hexagon), which is equal to a hex /3 ½ =4.0/3 ½ =2.3 nm for compound 2a , is indeed comparable to the length of the rigid bolaamphiphilic core L =2 L A + L B =2.1 nm as measured between the ends of the terminal glycerol groups, see Supplementary Fig. S10 . As a unit cell consists of just one hexagonal cylinder, all cylinders contain both R F and R H side chains. The ED map ( Fig. 3a ) suggests, however, that there is local core-shell phase separation within a cylinder, with the electron-rich fluorinated groups clustering in the centre (purple), and the aliphatic groups (red) located close to the terphenyl walls (green). We can define a reduced area per molecule A ′ as the volume of the columnar phase per molecule divided by the average spacing between the molecules along the column axis. Simply, A ′= A unitcell / j =3 ½ a hex 2 /2 j , where j is the number of cylinder walls per unit cell, that is, j =3 in the case of the Col hex phase. For compound 2a A ′=4.6 nm 2 ( Supplementary Table S6 ). 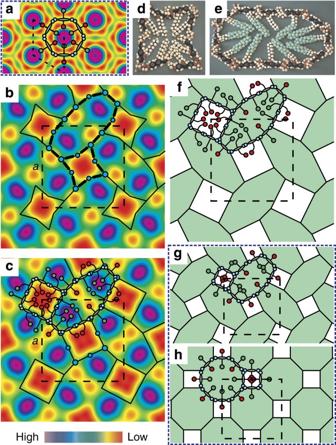The values of A ′ will be used in the next section. Figure 3: Electron density (ED) maps and phase structures. (a) ED map of the hexagonal columnar phase with core-shell structure of compound2a. (b,c) ED maps of compounds1aand1dreconstructed from the diffraction patterns inFig. 2candSupplementary Fig. S7c, respectively—for details seeSupplementary MethodsandSupplementary Fig. S11. Black lines inband grey ellipses ina,c,f,gandhmark the positions of terphenyl cores, blue dots are glycerol groups, and red and green dots ina,c,f,g,hare, respectively,RHandRFside chains. (d,e) CPK models of a stratum of the square and octagonal cylinders, respectively, for compound1a(the remaining space indandeis filled by chains from the lower and upper strata). (f) Representation of the giant octagon/squarep4gmhoneycomb as a two-colour tiling—cf.Fig. 1. (g,h) Hypothetical alternative octagon/square tilings with single-molecule wall lengths; plane groups (g)p4gm, (h)p4mm; in both cases overcrowding of the small squares with four long alkyl chains is evident. Figure 3: Electron density (ED) maps and phase structures. ( a ) ED map of the hexagonal columnar phase with core-shell structure of compound 2a . ( b , c ) ED maps of compounds 1a and 1d reconstructed from the diffraction patterns in Fig. 2c and Supplementary Fig. S7c , respectively—for details see Supplementary Methods and Supplementary Fig. S11 . Black lines in b and grey ellipses in a , c , f , g and h mark the positions of terphenyl cores, blue dots are glycerol groups, and red and green dots in a , c , f , g , h are, respectively, R H and R F side chains. ( d , e ) CPK models of a stratum of the square and octagonal cylinders, respectively, for compound 1a (the remaining space in d and e is filled by chains from the lower and upper strata). ( f ) Representation of the giant octagon/square p 4 gm honeycomb as a two-colour tiling—cf. Fig. 1 . ( g , h ) Hypothetical alternative octagon/square tilings with single-molecule wall lengths; plane groups ( g ) p 4 gm , ( h ) p 4 mm ; in both cases overcrowding of the small squares with four long alkyl chains is evident. Full size image Structure of the p 4 gm phase in compounds 1 The lattice parameter a squ of the Col squ / p 4 gm phase ( a squ =9.37–9.83 nm) is almost five times larger than the length L of the bolaamphiphilic core ( L =2.1 nm), suggesting a very different and more complex structure than observed for compounds 2 . Further information was gained from ED maps, reconstructed from the small-angle X-ray scattering (SAXS) intensities of compound 1a with the shortest and compound 1d with the longest alkyl chain ( Fig. 3b,c ). The reconstruction procedure and the choice of phase combination are described in the Methods and Supplementary Information ( Supplementary Methods and Supplementary Fig. S11 ), respectively. The ED maps of 1a and 1d are similar, having two large square-shaped and four smaller circular low-ED regions (red) in each unit cell; these are attributed to areas occupied by the alkyl chains. In addition, there are four high-ED regions (blue/purple) attributed to the R F chains. The low-ED regions are larger for 1d than for 1a . This is in line with the increase in alkyl chain length from n =10 ( 1a ) to n =16 ( 1d ), giving support for the phase choice used in the ED reconstruction. The high- and low-ED areas are separated by a continuum of medium ED (green) formed primarily by the aromatic cores, the hydrogen-bonding networks and also by regions where R H and R F chains are mixed, giving a medium average ED. Based on the experimental results, the following packing model can be deduced. For 1d ( Fig. 3c ), the side length of the low-ED squares is ~4.0 nm, which is about twice the length of the bolaamphiphilic core. Hence, it seems that the alkyl chains are enclosed within walls of square-shaped cylinders with the sides containing two end-to-end H-bonded bolaamphiphiles in a line (referred to here as 'giant square' or 8-square cylinders). The second type of cylinders has a cross-section in the shape of a large elongated polygon with 12 molecules linked end-to-end along its circumference. The polygon can be regarded as a giant octagon, with successive sides containing 2,1,2,1,2,1,2,1 molecules in length ( Fig. 3c ). Thus, the honeycomb combines giant square and octagonal cylinders in a 1:1 ratio. The above model implies that the number of molecules in the cross-section of the unit cell is j =20. This is confirmed by dividing the area of the p 4 gm unit cell of compounds 1 with the molecular area A ′ derived from the comparison with the equivalent compounds 2 . The details of the calculation and correction for the small differences in molecular volume are given in the Methods and Supplementary Table S7 . The resulting average value of j is 19.2 in the Col squ / p4gm phase of compounds 1 ( Supplementary Table S8 ), thus indeed supporting the above giant octagon/square model of the phase. By applying the above comparison between compounds 1 and 2 , we have avoided the necessity of not only measuring densities, but also of making an arbitrary estimate of the value of the intermolecular spacing along the column. Nevertheless, we have actually measured the room-temperature density of compound 1a as 1.43 g cm −3 . Using this value and the unit cell area, A =87.80 nm 2 , for 20 molecules per unit cell, we obtain the average intermolecular distance projected on the cylinder axis as c =0.34 nm (where c =20 M /( N A Aρ ), where M is the molecular weight (1,284 g/mol). Note that c is somewhat underestimated as the density at the temperature of the LC will be lower than 1.43 g cm −3 measured at room temperature. According to our ED-backed model of the p 4 gm honeycomb, the alkyl chains fill the square cylinders ( Fig. 3d ) and the R F chains occupy the majority of the space inside the octagonal cylinders ( Fig. 3e ). However, as 4 out of 12 octagon-forming molecules lie on the boundary between two octagons ( Fig. 3b,c,f ), their alkyl chains must be incorporated into the octagons. These alkyls form additional low-ED regions (red) inside the octagonal cylinders and divide the R F domains into two distinct R F -rich high-ED columns (blue/purple). Hence, the structure is made up of two different types of giant cylinders and it simultaneously combines intercolumnar with intracolumnar segregation. Notably, the intracolumnar segregation in the giant 12-octagons, cutting the R F region in half, differs from the usually observed simple core-shell structures, such as in the hexagonal honeycomb of compounds 2 ( Fig. 3a ), or in similar systems observed previously [34] . Bendy walls and surface anchoring For compound 1a ( Fig. 3b ) with alkyl chains much shorter than those in 1d , the walls of the giant square alkyl cylinder probably bend inwards, leading to a distortion into four-arm star shape. This simultaneously modifies the shape of the octagons, which can now be considered as dodecagons. It seems that the flexibility of the giant squares with hydrogen-bonded hinges in the middle of each side, allows the precise adoption of the polygon size and shape required. This seems to be the key to the stability of the Col squ / p 4 gm phase over a wide range of alkyl chain lengths (decyl to hexadecyl) and over a fairly wide temperature interval. Returning to the GISAXS pattern in Fig. 2d , there must be a reason for the two distinct orientations of the reciprocal lattice observed, that is, for the honeycomb to lie either with one of its {100} or {210} planes on the flat substrate (three Miller indices are used in this paragraph to highlight the 3D bulk nature of the phase). In fact, a third orientation, {110}, is also frequently seen ( Supplementary Fig. S8 ). As observed previously [35] , if lying with their long axis parallel to the substrate (planar anchoring), the cylinders choose to lie on a side that maximizes their polar groups' contact with the polar substrate. 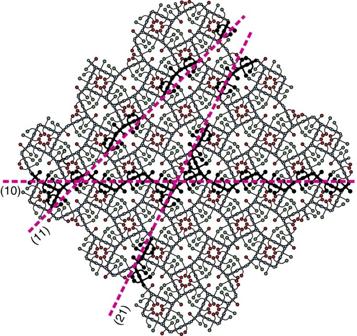At the same time, the contact with the substrate should cause minimum lattice distortion. Figure 4: Substrate contact planes. View of the Colsqu/p4gmhoneycomb along the cylinder axis with the projections of the three planes preferred for contact with the substrate (dashed purple lines). The molecules likely to lie on the substrate, after local adjustment of the lattice, are highlighted. Figure 4 shows the projections of the three hk 0 planes preferred by the substrate. The highlighted molecules require relatively minor adjustment to lie flat on the substrate. Notably, the {110} and {210} planes, as drawn in Fig. 4 , bridge the gap across the octagonal cylinders. It seems plausible that surface reconstruction occurs on the above { hk 0} planes when in contact with the substrate, cutting the octagons in half by adding extra bridging molecules. In the bulk, however, bridging the octagons is unlikely, as this would require the unit cell to contain more than the calculated j =20 molecules. Thus, the observed alignment behaviour is fully in line with the proposed LC phase structure. Figure 4: Substrate contact planes. View of the Col squ / p 4 gm honeycomb along the cylinder axis with the projections of the three planes preferred for contact with the substrate (dashed purple lines). The molecules likely to lie on the substrate, after local adjustment of the lattice, are highlighted. Full size image Comparing compounds 1b and 2a , 1c and 2b and so on, illustrates how the replacement of only four hydrogens by fluorines increases the incompatibility between the R F and R H chains sufficiently to cause their separation into distinct cylinders, smaller square shaped for R H and larger octagonal mainly for R F . The difference in cylinder shape is a result of unequal effective volumes of the two chains. A different scenario has been described recently for similar terphenyl-based X-shaped amphiphiles, where the fluorinated chains were shorter and instead of alkyls, the non-fluorinated side chains were larger-sized carbosilanes [26] . The overall side-chain volume was similar to that in the present compounds, but the side-chain effective volumes were more closely matched. Hexagonal honeycombs were formed and the area per molecule was as here, 4.7 nm 2 . At higher temperatures, the two side-chain types shared the same cylinders, as here in compounds 2 ( Fig. 3a ). However, at lower temperatures, a Curie-type transition led to a superlattice phase with the hexagonal cell walls fully preserved, but with the chains redistributed to give pure carbosilane and mixed carbosilane-fluorinated cells in a 1:2 ratio (see Fig. 1d ). Both, this low-temperature hexagonal phase and the current octagon–square phase are frustrated by geometry and incomplete phase separation, yet only for compounds 1a – 1d a large-cell honeycomb with cylinders of very different shape and size is obtained. It may be surprising to find only giant long-wall cylinders in the present p 4 gm phase, although there would be enough space to accommodate the fluorinated chains in short-walled eight-octagons, as in the small-cell p 4 gm structure in Fig. 3g , or even in the theoretically predicted [36] p 4 mm structure containing regular eight-octagon ( Fig. 3h ), where the R F chains would also be able to reach the column centre. However, what seems to prevent the formation of these simpler structures is the overcrowding that would result in the small alkyl-filled square columns. With compounds 1a – 1d a degree of complexity of fluid LC superstructures was achieved that is unique in soft self-assembled chemical systems. We note that a structure similar to the present octagon–square honeycomb has been observed recently in zeolitic imidazolate framework crystals, although that is a 3D solid-state structure and is on an atomic rather than mesoscopic length scale [37] . To the best of our knowledge, these are the largest polygonal cylinders observed so far, exceeding even those obtained with considerably larger molecules [15] , and were achieved by a combination of frustrated space-filling and frustrated microphase separation in soft self-assembly. The flexibility of the cylinder walls is believed to provide extra stability and versatility of the structure. Moreover, a unique combination of intercolumnar and complex intracolumnar segregations was obtained, establishing a new level of complexity in LC design. Synthesis All compounds were synthesized in-house according to the synthetic procedure shown in Fig. 5 . Details of the synthesis and the analytical data of compounds 1a – 1d and 2a are given in the accompanying Supplementary Methods . Optical microscopy Phase transitions were determined by polarizing optical microscopy (Optiphot 2, Nikon) in conjunction with a heating stage (FP 82 HT, Mettler) and by differential scanning calorimetry (DSC-7, Perkin-Elmer) at heating/cooling rates of 10 K min −1 . X-ray diffraction The SAXS experiments were carried out at station I22, Diamond Light Source. The wavelength used was 1 Å. Two-dimensional SAXS patterns were recorded using a Rapid II area detector, and converted to 1-d curves by azimuthal averaging. Positions and intensities of the diffraction peaks were measured using PeakSolve (Galactic). GISAXS experiments were performed on station BM28 (XMaS line) at European Synchrotron Radiation Facility (ESRF) and on beamline I07 at Diamond Light source. Thin-film samples were prepared from the melt on a silicon wafer. The film-coated Si plates of 5×5 mm 2 were placed on top of a custom built heater, which was then mounted on a six-circle goniometer. A MarCCD 165 detector was used at ESRF and Pilatus 2M (Dectris) detectors were used at Diamond. The sample enclosure and the beam pipe were flushed with helium. Aligned samples for wide-angle X-ray diffraction were obtained on a glass plate by slow cooling (1–0.01 K min −1 ) of a small droplet. The aligned samples were held on a temperature-controlled heating stage and the diffraction patterns were recorded with a 2D detector (HI-STAR, Siemens). Reconstruction of ED maps As is well known, diffraction intensities are related to the ED distribution E ( x , y ) by Fourier transformation. For two-dimensional structures, we have Here F ( hk ) is the structure factor of a diffraction peak with index ( hk ). It is related to the experimentally observed diffraction intensity through Here K is a constant related to the sample volume, incident beam intensity and so on. In this paper, we are only interested in relative EDs, hence this constant is simply taken to be 1. Thus, the ED is In general, the structure factor F ( hk ) is a complex number, so the phase angle φ ranges from 0 to 2 π . The phase angle φ cannot be determined directly from diffraction experiments. However, for centro-symmetric structures, such as the ones in this work, the problem is considerably simplified by the fact that F ( hk ) is a real number and the phase angle φ can only take up the values of 0 or π . For LC systems, where the number of observed reflections is limited, this allows one to examine all possible phase combinations, and the choice of a combination can be made on the merit of each reconstructed ED maps, combined with the additional knowledge of the molecules (molecular shape, length, volume of each part and the distribution of ED among the different moieties). Investigation of homologous series of compounds with varying size of a particular group is especially helpful in determining the phase combination. The details of the phase choice in this work are given in Supplementary Methods , including Supplementary Fig. S11 . Calculation of the number of molecules per unit cell ( j ) If the structure was 3D ordered, we could calculate j from measured density and the calculated unit cell volume. However, with there being no long-range order along the column axis, the average spacing c between adjacent molecules in the stack could not be determined by diffraction. Therefore, we resort to comparing compounds 1 in the p 4 gm phase with compounds 2 in the p 6 mm phase; in the latter phase j is known to be 3 and, as the unit cell area is known, the area per molecule A ′ is known precisely—see Supplementary Table S6 . In determining A ′ for the p 4 gm phase of compounds 1 , we rely on the assumption that c is similar in those compounds 1 and 2 that have similar molecular volumes. Thus, we compare 1a with 2b , 1b with 2c and 1c with 2d and apply an additional correction for the small difference in molecular volumes between 1a and 2b , 1b and 2c and so on—see Supplementary Table S7 . The calculated molecular area A ′ for compounds 1 and the associated value of j are given in Supplementary Table S8 . How to cite this article: Liu, F. et al . Arrays of giant octagonal and square cylinders by liquid crystalline self-assembly of X-shaped polyphilic molecules. Nat. Commun. 3:1104 doi: 10.1038/ncomms2096 (2012).